High-resolution eye tracking using V1 neuron activity Studies of high-acuity visual cortical processing have been limited by the inability to track eye position with sufficient accuracy to precisely reconstruct the visual stimulus on the retina. As a result, studies of primary visual cortex (V1) have been performed almost entirely on neurons outside the high-resolution central portion of the visual field (the fovea). Here we describe a procedure for inferring eye position using multi-electrode array recordings from V1 coupled with nonlinear stimulus processing models. We show that this method can be used to infer eye position with 1 arc-min accuracy—significantly better than conventional techniques. This allows for analysis of foveal stimulus processing, and provides a means to correct for eye movement-induced biases present even outside the fovea. This method could thus reveal critical insights into the role of eye movements in cortical coding, as well as their contribution to measures of cortical variability. Studies of high-acuity visual processing in awake animals are invariably faced with the difficulty of accounting for the effects of eye movements on the retinal stimulus. Animals that are well-trained to maintain precise fixation continuously make involuntary eye movements, composed of both microsaccades and drift [1] . Even in anaesthetized and paralysed animals, the eyes undergo slow drifts, as well as movements tied to heartbeat and respiration [2] . The resulting uncertainty in the retinal stimulus can be large relative to the fine receptive fields (RFs) of neurons in primary visual cortex (V1), which are fixed in retinotopic coordinates [3] , [4] , [5] , [6] . Conventional eye-tracking methods, such as implanted scleral eye coils [7] and optical tracking techniques [8] , have accuracies comparable to the magnitude of the fixational eye movements themselves (about 0.1°) [1] , [5] , [6] , [9] , making them ill-suited to correct for such fine-grained changes in eye position. Thus, without accurately accounting for eye movements, the stimulus presented to such neurons is both uncontrolled and unknown, greatly limiting analyses of neural stimulus processing, cortical variability and the role of eye movements in visual processing. This is especially true for V1 neurons representing the central portion of the visual field (the fovea), which have extremely small RFs. As a result, relatively little is known about whether they process visual stimuli differently from neurons representing the non-foveal visual field, which is an important question given the overrepresentation of the fovea throughout visual cortex [10] and the critical role the fovea has in a variety of high-acuity visual behaviours [11] . Although basic tuning properties of foveal V1 neurons have been measured [12] , [13] , the detailed functional descriptions of V1 stimulus processing that have been developed for parafoveal neurons [14] , [15] , [16] have yet to be tested, and important questions about functional specialization in the fovea remain [17] , [18] , [19] , [20] . To address these problems, here we present a method for inferring an animal’s eye position using the activity of the V1 neurons themselves, leveraging their finely tuned RFs to derive precise information about the position of the stimulus on the retina. Our method utilizes multi-electrode recordings and a recently developed nonlinear modelling approach [21] , [22] , [23] , [24] to estimate an animal’s eye position, along with its associated uncertainty, at the high spatial and temporal resolutions needed to study foveal V1 neurons. We demonstrate this approach using multi-electrode array recordings from awake behaving macaques, and show that it allows for estimation of eye position with an accuracy on the order of 1 min of arc (~0.017°). Our method yields eye-tracking improvements in both foveal and parafoveal recordings, and is robust to the number and composition of the recorded units. Using this method allows us to obtain detailed functional models of the stimulus processing of foveal V1 neurons that are otherwise largely or entirely obscured by eye movements. In addition to allowing detailed analyses of high-resolution stimulus processing, our method can identify and correct for the effects of eye movements on measures of cortical variability, which has important implications for studies of neural coding more generally [25] , [26] , [27] . Inferring eye position using stimulus processing models To illustrate the profound impact of fixational eye movements on estimates of foveal neuron stimulus processing, we consider a simulated V1 ‘simple cell’ whose RF (a Gabor function) has a preferred spatial frequency typical of foveal neurons (5 cyc deg −1 ) [12] , [13] , [28] , which is presented with random bar patterns at the model neuron’s preferred orientation ( Fig. 1a–c ). Were the animal to maintain perfect fixation, the spatial structure of its RF could easily be inferred from its spiking activity. However, because the response of a neuron to a given displayed stimulus is highly sensitive to the precise position of the eye along the axis orthogonal to the bars, such RF estimation fails in the presence of fixational eye movements ( Fig. 1c ). 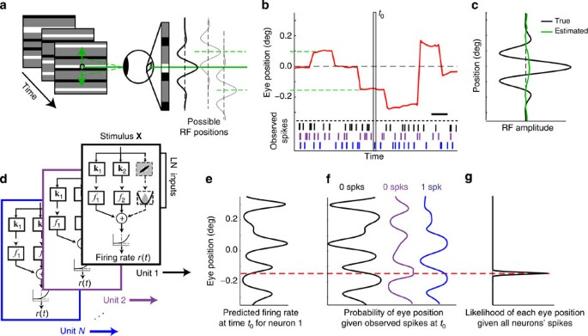Figure 1: Inferring eye position using neural activity. (a) We present a 100-Hz random bar stimulus (left). Small changes in eye position shift the image on the retina, causing changes in the visual input that are large relative to the receptive fields of typical foveal neurons (right). (b) An example eye position trace (red) demonstrating the typical magnitude of fixational eye movements relative to the fixation point (0°), using the same vertical scale asa. Scale bar, 200 ms. (c) Estimation of the 1-D receptive field profile (green) for a simulated example neuron (preferred spatial frequency=5 cyc deg−1) is entirely obscured when fixational movements are not accounted for (true profile in black). (d) Quadratic stimulus processing models were fit to each recorded unit. The quadratic model is specified by a set of stimulus filters associated with linear and quadratic transforms, whose outputs are summed together and passed through a spiking nonlinearity to generate a predicted firing rate. (e) At a given timet0(vertical box inb), each model can be used to predict the firing rate of each neuron as a function of eye position (shown for an example neuron). (f) The observed spike counts att0can be combined with the model predictions to compute the likelihood of each eye position from each model (for example, black, purple, blue). For the case shown, the observation of 0 spikes (black neuron) implies a higher probability of eye positions associated with low firing rates (black, left). (g) Evidence is accumulated across neurons by summing their log-likelihood functions, and is integrated over time, resulting in an estimate of the probability of each eye position (black) that is tightly concentrated around the true value (dashed red). Figure 1: Inferring eye position using neural activity. ( a ) We present a 100-Hz random bar stimulus (left). Small changes in eye position shift the image on the retina, causing changes in the visual input that are large relative to the receptive fields of typical foveal neurons (right). ( b ) An example eye position trace (red) demonstrating the typical magnitude of fixational eye movements relative to the fixation point (0°), using the same vertical scale as a . Scale bar, 200 ms. ( c ) Estimation of the 1-D receptive field profile (green) for a simulated example neuron (preferred spatial frequency=5 cyc deg −1 ) is entirely obscured when fixational movements are not accounted for (true profile in black). ( d ) Quadratic stimulus processing models were fit to each recorded unit. The quadratic model is specified by a set of stimulus filters associated with linear and quadratic transforms, whose outputs are summed together and passed through a spiking nonlinearity to generate a predicted firing rate. ( e ) At a given time t 0 (vertical box in b ), each model can be used to predict the firing rate of each neuron as a function of eye position (shown for an example neuron). ( f ) The observed spike counts at t 0 can be combined with the model predictions to compute the likelihood of each eye position from each model (for example, black, purple, blue). For the case shown, the observation of 0 spikes (black neuron) implies a higher probability of eye positions associated with low firing rates (black, left). ( g ) Evidence is accumulated across neurons by summing their log-likelihood functions, and is integrated over time, resulting in an estimate of the probability of each eye position (black) that is tightly concentrated around the true value (dashed red). Full size image Our model-based approach leverages the spatial sensitivity of V1 neurons to infer the precise position of the stimulus on the retina (and hence the direction of gaze). We use models of each neuron's stimulus processing ( Fig. 1d ) to estimate, at each time, the dependence of the neuron's firing rate on eye position ( Fig. 1e ). The observed spiking of the neuron can then be used to compute the likelihood of each eye position ( Fig. 1f ) [5] , [29] , [30] . Although the evidence for eye position provided by a single neuron at a given time is typically very weak, we can obtain precise and robust eye position estimates by integrating such information over a population of recorded neurons ( Fig. 1g ), and by using the fact that eye position changes slowly across time, except during microsaccades. This method can also naturally incorporate information from hardware eye-tracking to provide additional evidence about the eye position (see Methods), although we do not do so when comparing inferred and coil-measured eye positions to allow for unbiased validation. A key element of this procedure is the ability to construct models that accurately predict the responses of V1 neurons to arbitrary stimuli. To this end, we used a probabilistic modelling framework that describes a neuron's spiking response as a cascade of linear and nonlinear transformations on the stimulus ( Fig. 1d ) [21] , [22] , [23] , [24] . As illustrated in the preceding example, however, accurate models of foveal stimulus processing require detailed knowledge of the eye position ( Fig. 1c ). Our method thus utilizes an ‘expectation-maximization (EM)’ algorithm that iterates between estimating the stimulus processing models given estimates of eye position and estimating the sequence of eye positions given the stimulus processing models. In using a probabilistic framework that considers all possible eye positions, the approach also provides continuous estimates of eye position uncertainty, unlike any previous eye-tracking methods. Precision and accuracy of the inferred eye positions We first demonstrate this approach using the activity of foveal V1 neurons (0.4–0.8° eccentricity) recorded from an awake macaque during simple fixation tasks using a 96-electrode planar ‘Utah’ array. During these tasks, the animal was presented with a ‘ternary noise’ stimulus, consisting of random patterns of horizontal black and white bars updated at 100 Hz, while eye position was monitored with a scleral search coil. We then used our method to infer the vertical component of eye position given the observed spiking activity on the array. The inferred eye positions were remarkably precise ( Fig. 2a ), with estimated uncertainties (s.d. of posterior distribution) typically less than 1 arc-min (median uncertainty 0.51±0.052 arc-min; mean±s.d. across N =8 recordings). These uncertainty estimates reflect the strength of evidence that is provided by observed neural activity at each time, and closely match the distribution of errors between inferred and ‘ground truth’ eye positions in simulations ( Supplementary Fig. 1 ). Thus, by integrating information over many neurons (as well as using information about the eye movement dynamics), our algorithm is able to achieve much finer precision than the spatial scale of individual neurons’ RFs (with features on the order of 0.1° or 6 arc-min), and even smaller than the visual angle subtended by individual pixels in the display (1.1 arc-min). 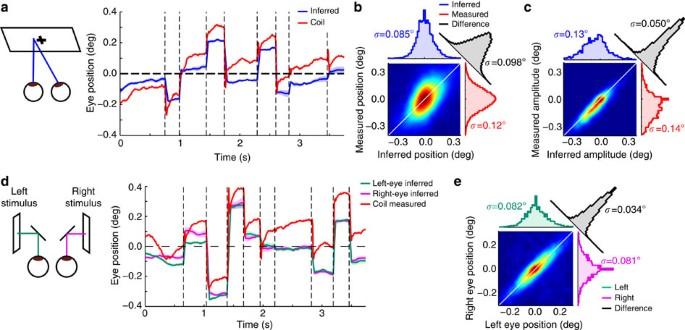Figure 2: Validation of inferred eye positions. (a) An example inferred conjugate eye position (blue), compared with the eye position measured using the eye coil (red). The shaded blue region (mean±s.d.) shows the model-based estimate of uncertainty. (b) The joint probability distribution of inferred (horizontal axis) and coil-measured (vertical axis) eye positions for an example recording, demonstrating substantial differences between the two signals. As a result, the distribution of their differences (black) had a similar width to their marginal distributions (red, blue). Colour is scaled to represent the square-root of the joint probability for visualization. (c) In contrast, the inferred and coil-measured microsaccade amplitudes were strongly correlated, as shown by the much narrower joint distribution measured for the same recording as inb. (d) We also made independent estimates of both eye positions by presenting a different stimulus to each eye (left). Example trace showing separately inferred left (green) and right (magenta) eye positions, compared with the coil measurement (red). (e) Inferred left and right eye positions were in close agreement, as demonstrated by the joint, marginal and difference distributions, shown as inb,c. Figure 2: Validation of inferred eye positions. ( a ) An example inferred conjugate eye position (blue), compared with the eye position measured using the eye coil (red). The shaded blue region (mean±s.d.) shows the model-based estimate of uncertainty. ( b ) The joint probability distribution of inferred (horizontal axis) and coil-measured (vertical axis) eye positions for an example recording, demonstrating substantial differences between the two signals. As a result, the distribution of their differences (black) had a similar width to their marginal distributions (red, blue). Colour is scaled to represent the square-root of the joint probability for visualization. ( c ) In contrast, the inferred and coil-measured microsaccade amplitudes were strongly correlated, as shown by the much narrower joint distribution measured for the same recording as in b . ( d ) We also made independent estimates of both eye positions by presenting a different stimulus to each eye (left). Example trace showing separately inferred left (green) and right (magenta) eye positions, compared with the coil measurement (red). ( e ) Inferred left and right eye positions were in close agreement, as demonstrated by the joint, marginal and difference distributions, shown as in b , c . Full size image Although the inferred eye positions exhibited qualitatively similar dynamics to those measured using the coil ( Fig. 2a ), the absolute differences between the two eye position signals were substantial ( Fig. 2b ). The fact that these differences are consistent with previous estimates of eye coil accuracy [5] , [9] , combined with several lines of evidence described below, strongly suggests that the discrepancies are largely due to inaccuracies in the coil measurements. Despite the disagreement between coil- and model-based estimates of absolute eye position, changes in eye position over shorter time scales, such as microsaccade amplitudes, were in close agreement ( Fig. 2c ). This agreement of inferred and measured microsaccade amplitudes not only provides validation of the inferred eye positions but also suggests that such reliable short-timescale measurements from the eye coil can be integrated into our inference procedure to provide additional eye position information (see Methods). To further validate the accuracy of the model-based eye position estimates, we used a haploscope to present binocularly uncorrelated stimuli, and made independent estimates of the left and right eye positions ( Fig. 2d ; see Methods). Because the animal's vergence is expected to be very precise [5] , [6] , [31] , differences between the inferred left and right eye positions can be used to place an upper bound on the error in our eye position estimates. Note that this upper bound is conservative, both because some differences are expected due to real vergence fluctuations, and because only half of the stimulus was utilized to infer each eye position. Nevertheless, we found that the inferred left and right eye positions were in agreement to within about 2 arc-min ( Fig. 2e ), comparable to previous estimates of vergence error [5] , [6] , [31] . Assuming the left and right eye position errors are uncorrelated, this suggests an upper bound of 1.4 arc-min for the accuracy of inferred eye positions (removing a factor of square-root of two). Estimation of detailed functional models Our model-based inference procedure also involves (and depends on) the estimation of detailed functional models of V1 neurons. To model both ‘simple’ and ‘complex’ cell stimulus processing parsimoniously, we utilized a quadratic cascade model whose response is calculated as a sum over a set of linear and squared stimulus filters [22] , [24] . Such a model often captures many elements of a given neuron’s stimulus processing even without using eye position information (that is, assuming perfect fixation; Fig. 3a , left). However, using the stimulus corrected for the estimated eye positions usually results in a dramatic sharpening of the linear stimulus filter, along with more modest changes to the squared components of the model ( Fig. 3a , right). 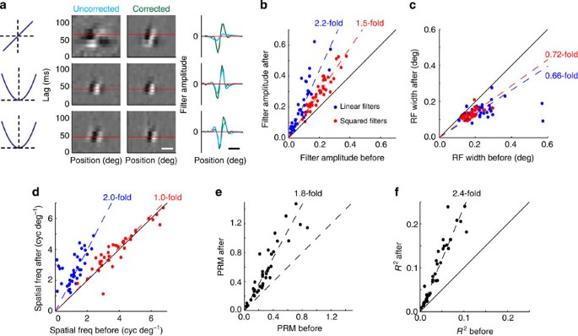Figure 3: Improvement in model fits after correcting for eye movements. (a) The quadratic model of an example single-unit before (left) and after (right) correcting for eye movements. Spatiotemporal filters are shown for the linear term (top) and two quadratic terms (bottom), with the greyscale independently normalized for each filter. The spatial tuning of each filter (at the optimal time lag shown by the horizontal red lines) is compared before (cyan) and after (green) eye position correction, clearly demonstrating the large change in the linear filter, and smaller changes in the quadratic filters. Horizontal scale bar is 0.2°. (b) Amplitudes of the linear (blue) and squared (red) stimulus filters across all single units (N=38) were significantly higher after correcting for eye position. (c) Correcting for eye position decreased the apparent widths of linear and squared stimulus filters. (d) The preferred spatial frequency of linear stimulus filters increased greatly with eye correction, whereas it changed little for the squared filters. (e) Spatial phase-sensitivity of neurons, measured by their phase-reversal modulation (PRM; see Methods), increased substantially after correcting for eye movements. (f) Model performance (likelihood-basedR2) increased by over two-fold after correcting for eye movements. Note that we use a leave-one-out cross-validation procedure (see Methods) when estimating all the above model changes with eye corrections. Figure 3: Improvement in model fits after correcting for eye movements. ( a ) The quadratic model of an example single-unit before (left) and after (right) correcting for eye movements. Spatiotemporal filters are shown for the linear term (top) and two quadratic terms (bottom), with the greyscale independently normalized for each filter. The spatial tuning of each filter (at the optimal time lag shown by the horizontal red lines) is compared before (cyan) and after (green) eye position correction, clearly demonstrating the large change in the linear filter, and smaller changes in the quadratic filters. Horizontal scale bar is 0.2°. ( b ) Amplitudes of the linear (blue) and squared (red) stimulus filters across all single units ( N =38) were significantly higher after correcting for eye position. ( c ) Correcting for eye position decreased the apparent widths of linear and squared stimulus filters. ( d ) The preferred spatial frequency of linear stimulus filters increased greatly with eye correction, whereas it changed little for the squared filters. ( e ) Spatial phase-sensitivity of neurons, measured by their phase-reversal modulation (PRM; see Methods), increased substantially after correcting for eye movements. ( f ) Model performance (likelihood-based R 2 ) increased by over two-fold after correcting for eye movements. Note that we use a leave-one-out cross-validation procedure (see Methods) when estimating all the above model changes with eye corrections. Full size image Across the population, adjusting the stimulus to correct for inferred eye positions resulted in large changes in the estimated properties of V1 neurons, including their spatial tuning widths, preferred spatial frequencies and the magnitudes of their stimulus filters ( Fig. 3b–d ). Much larger changes were observed in the linear filters compared with the quadratic filters, because the quadratic filters are less sensitive to small displacements of the stimulus [32] , and thus are closer to the ‘true filters’ before correcting for eye movements. As a result of this differential sensitivity of linear and quadratic terms to eye movement corrections, estimates of the spatial phase sensitivity of neurons (similar to F1/F0, ref. 33 ) increased by 1.8-fold after correcting for eye movements ( Fig. 3e ; see Methods), suggesting that phase-invariance of V1 neurons could be dramatically over-estimated when eye position corrections are not performed. Note that these tuning properties (as well as others) can be derived from the eye position-corrected models to provide analogues of standard ‘tuning curve’ measurements that are unbiased by the effects of eye movements. These changes in model properties also resulted in large improvements in model performance, which we evaluated using the likelihood-based R 2 (ref. 34 ). Measurements of R 2 were applied to each model neuron using a ‘leave-one-out’ cross-validation procedure, where the neuron being considered was not used for estimating eye position (see Methods). R 2 values for our models increased by 2.4-fold after correcting for inferred eye positions ( Fig. 3f ), suggesting that a majority of the information being conveyed by these neurons was in fact being missed when our models did not take into account the fixational eye movements. In contrast, when we used the coil measurements to correct for eye position, we did not observe significant improvements in model fits compared with assuming perfect fixation ( Supplementary Fig. 2 ) [5] , [35] . This highlights an additional advantage of a model-based approach: the stimulus processing models themselves provide a means to objectively compare the accuracy of different eye position estimates, using the observed neural activity as evidence. Two-dimensional eye position inference and model estimation Although we have thus far demonstrated the use of our method for inferring a single dimension of eye position, it is straightforward to extend the procedure to infer the full two-dimensional eye position. In doing so, one necessarily introduces additional complexity to the underlying stimulus processing models and/or eye position estimation procedure (see Methods). Here we suggest two possible approaches that focus on different tradeoffs in this respect. One approach, which utilizes relatively simple stimulus processing models, is to interleave stimuli composed of horizontal and vertical bar patterns ( Fig. 4a ), using each stimulus orientation to infer the orthogonal component of eye position. Indeed, we find that this straightforward extension allows us to simultaneously infer both dimensions of eye position ( Fig. 4b ) with comparable results to those described above. 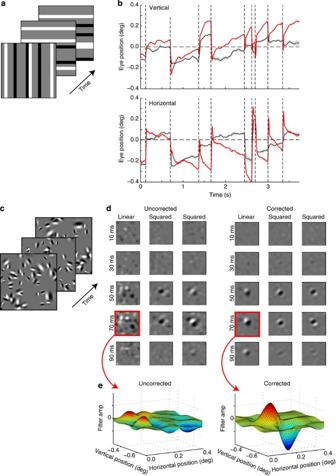Figure 4: Two-dimensional (2D) eye position inference. (a) Schematic of the ternary noise stimulus with randomly interleaved horizontal and vertical bar orientations. (b) Inferred vertical (top) and horizontal (bottom) eye positions (black) using the stimulus shown ina, compared with coil-measured eye positions (red). (c) Schematic of the sparse Gabor noise stimulus used to estimate full spatiotemporal models. (d) Spatiotemporal stimulus filters estimated for an example single unit before (left) and after (right) correcting for eye position, showing clear sharpening of spatial profiles with 2D eye correction. Each filter is shown as a sequence of spatial profiles across time lags. (e) Spatial profiles of the uncorrected (left) and corrected (right) linear stimulus filters at the neuron's optimal time lag (70 ms). Figure 4: Two-dimensional (2D) eye position inference. ( a ) Schematic of the ternary noise stimulus with randomly interleaved horizontal and vertical bar orientations. ( b ) Inferred vertical (top) and horizontal (bottom) eye positions (black) using the stimulus shown in a , compared with coil-measured eye positions (red). ( c ) Schematic of the sparse Gabor noise stimulus used to estimate full spatiotemporal models. ( d ) Spatiotemporal stimulus filters estimated for an example single unit before (left) and after (right) correcting for eye position, showing clear sharpening of spatial profiles with 2D eye correction. Each filter is shown as a sequence of spatial profiles across time lags. ( e ) Spatial profiles of the uncorrected ( left ) and corrected ( right ) linear stimulus filters at the neuron's optimal time lag (70 ms). Full size image A second approach uses more complex two-dimensional stimuli (such as ‘sparse Gabor noise’, Fig. 4c ), allowing for estimation of more sophisticated spatiotemporal models along with two-dimensional eye position. This approach necessarily requires more data for accurate parameter estimates, but produces models composed of stimulus filters with two spatial dimensions and one temporal dimension ( Fig. 4d ). For an example neuron, incorporating the inferred (two-dimensional) eye positions reveals a clear linear stimulus filter that was absent when fixational eye movements were ignored ( Fig. 4e ). This example thus illustrates both the feasibility and the potential importance of using our eye position inference method when analysing general spatiotemporal stimulus processing in V1. In fact, accurate eye position estimates are likely to be even more important when analysing two-dimensional stimulus processing, where the responses of neurons are sensitive to fluctuations along both spatial dimensions. Robustness to the size of the recoded neural population Although thus far we have utilized neural populations of ~100 units to infer eye position, this approach can also be applied with many fewer simultaneously recorded neurons. Using random sub-populations of various sizes, we found that the inferred eye positions were relatively insensitive to the size of the neural ensemble used, with accurate eye positions ( Fig. 5 ) even with ensembles as small as 10 units. Importantly, very similar results were obtained when using only ‘multi-unit’ activity to perform eye position inference, demonstrating that this often un-utilized element of multi-electrode recordings could serve to provide precise measurement of eye position on its own. 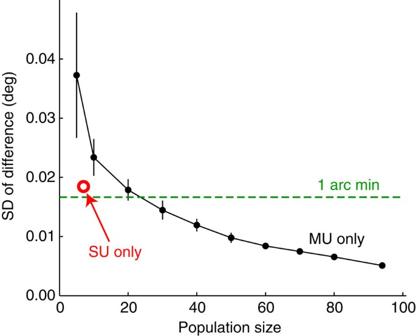Figure 5: Dependence of eye position inference on neural population size and composition. To determine how the results of our eye-tracking method depend on the size of the neural ensemble used, we ran our algorithm using randomly sampled (without replacement) sub-populations of units from an example array recording. When using only multi-units (black trace; error bars show mean±s.d.;N=15 sub-populations), the estimated eye positions were very similar (measured by the s.d. of the difference) to those obtained using both single-units and multi-units (SUs+MUs;N=101), even for relatively small populations. When using only the SUs (N=7; red circle), eye position estimates were even more similar to the best estimate compared with the equivalently sized population of MUs. Figure 5: Dependence of eye position inference on neural population size and composition. To determine how the results of our eye-tracking method depend on the size of the neural ensemble used, we ran our algorithm using randomly sampled (without replacement) sub-populations of units from an example array recording. When using only multi-units (black trace; error bars show mean±s.d. ; N =15 sub-populations), the estimated eye positions were very similar (measured by the s.d. of the difference) to those obtained using both single-units and multi-units (SUs+MUs; N =101), even for relatively small populations. When using only the SUs ( N =7; red circle), eye position estimates were even more similar to the best estimate compared with the equivalently sized population of MUs. Full size image The robustness of eye position inference to smaller numbers of recorded units was also tested using recordings made with 24-electrode linear probes. With the linear array, our eye position estimates again showed good agreement with the eye coil measurements ( Supplementary Fig. 3 ), and provided comparable improvements in model fits to those obtained with the planar array recordings (see below). Dependence on RF size across eccentricity The flexibility of acute laminar array recordings allowed us to gauge the impact of eye movements on neurons recorded from a range of foveal and parafoveal locations (~0.5–4° eccentricity). In fact, we found substantial model improvements for neurons throughout this range, which can be understood by considering the wide range of RF sizes present at a given eccentricity [28] , [36] , [37] ( Fig. 6a ). Indeed, the size of a neuron's RF largely determines how sensitive its response will be to eye position variability, and as a result, RF size is directly related to the magnitude of resulting model improvements after correcting for eye movements ( Fig. 6b ). 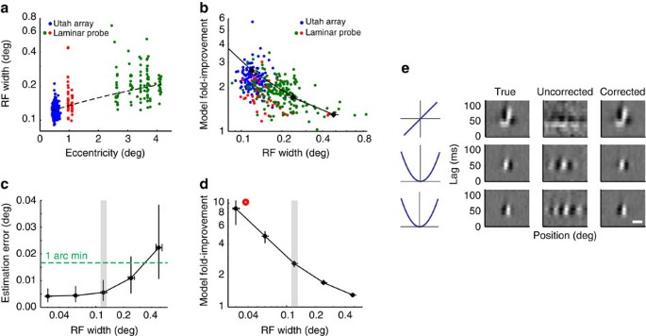Figure 6: Dependence of eye position and model estimation on RF size. (a) Recordings performed across different eccentricities showed a large range of RF widths at a given eccentricity, as well as the expected increase in average RF width with eccentricity. Each point represents the RF width and eccentricity of a given single- or multi-unit (N=76/274 SU/MU), colour-coded by electrode array and recording location (blue: Utah array, fovea,N=132; red: linear array, fovea,N=48; green: linear array, parafovea,N=170). The dashed line shows the linear fit between eccentricity and RF size (note semi-log axes). (b) Cross-validated improvements in model performance were larger for neurons with smaller RFs (correlation=−0.53,P=0). Units colour-coded as ina. A similar relationship was also found using simulated neural populations (see below: black trace). (c) Simulations, where ‘ground truth’ eye positions are known, were performed for V1 populations (N=101 units) having a range of RF widths. The accuracy of inferred eye positions increased for populations with smaller RFs, and remained below 1 arc-min even for populations with substantially larger RFs. Error bars show the median and inter-quartile range, and the RF widths of foveal neurons recorded on the planar array are indicated by the grey region. (d) For the same simulated V1 populations, improvements in model fits became more dramatic for neurons with smaller RFs, although they remained substantial even for neurons with much larger RFs. Note that this is the same trace as inb. (e) Stimulus filters can be recovered even for neurons with the smallest RF widths (left), as demonstrated for a simulated neuron with an RF width of 0.037° (red circle ind). Here, fixational eye movements almost entirely obscure the model estimates without eye position correction (that is, assuming perfect fixation; middle), but using the inferred eye positions recovers the structure of the neuron’s stimulus filters (right). Horizontal scale bar is 0.05°. Figure 6: Dependence of eye position and model estimation on RF size. ( a ) Recordings performed across different eccentricities showed a large range of RF widths at a given eccentricity, as well as the expected increase in average RF width with eccentricity. Each point represents the RF width and eccentricity of a given single- or multi-unit ( N =76/274 SU/MU), colour-coded by electrode array and recording location (blue: Utah array, fovea, N =132; red: linear array, fovea, N =48; green: linear array, parafovea, N =170). The dashed line shows the linear fit between eccentricity and RF size (note semi-log axes). ( b ) Cross-validated improvements in model performance were larger for neurons with smaller RFs (correlation=−0.53, P =0). Units colour-coded as in a . A similar relationship was also found using simulated neural populations (see below: black trace). ( c ) Simulations, where ‘ground truth’ eye positions are known, were performed for V1 populations ( N =101 units) having a range of RF widths. The accuracy of inferred eye positions increased for populations with smaller RFs, and remained below 1 arc-min even for populations with substantially larger RFs. Error bars show the median and inter-quartile range, and the RF widths of foveal neurons recorded on the planar array are indicated by the grey region. ( d ) For the same simulated V1 populations, improvements in model fits became more dramatic for neurons with smaller RFs, although they remained substantial even for neurons with much larger RFs. Note that this is the same trace as in b . ( e ) Stimulus filters can be recovered even for neurons with the smallest RF widths (left), as demonstrated for a simulated neuron with an RF width of 0.037° (red circle in d ). Here, fixational eye movements almost entirely obscure the model estimates without eye position correction (that is, assuming perfect fixation; middle), but using the inferred eye positions recovers the structure of the neuron’s stimulus filters (right). Horizontal scale bar is 0.05°. Full size image Conversely, the ensemble of RF sizes in a given recording will influence the accuracy of estimated eye positions, with ensembles consisting of smaller RFs providing more precise information about eye position. To systematically study the effects of RF size on the performance of our method, we simulated V1 responses to ternary noise stimuli during fixational eye movements, using populations of neurons that had the same properties as those recorded on the planar array but with their RFs scaled to larger and smaller sizes. By comparing the estimated eye positions and stimulus models to their simulated ‘ground truth’ values, we could then determine how the accuracy of our inferred eye positions, as well as their impact on model estimates, depended on the RF sizes of the underlying neural ensemble. As intuitively expected, neural ensembles with smaller RFs provided more accurate inferred eye positions ( Fig. 6c ) and improvements in model fits that were correspondingly more dramatic ( Fig. 6d ), because they were more sensitive to the precise eye position. Nevertheless, ensembles with larger RFs still yielded eye position estimates that were accurate to within 2 arc-min ( Fig. 6c ), with significant associated model improvements, suggesting that accounting for fixational eye movements is likely to be important even for V1 recordings outside the fovea [3] , [5] , [6] , [38] . In fact, the relationship between model improvements and RF sizes predicted by these simulations matched fairly closely with that observed in our data ( Fig. 6b ). These simulations also demonstrated that our method is able to robustly infer the true eye position even when using neurons with RFs four times smaller than those we recorded from the fovea. In this case, the eye position variability is much larger than the neurons' RFs ( Fig. 6e ), and as a result, the initial model estimates (assuming perfect fixation) were extremely poor ( Fig. 6e ). Nevertheless, the iterative inference procedure was able to recover the neurons' stimulus filters in addition to the ‘true’ eye position used for the simulation. The effects of eye movements on cortical variability The broad impact of eye movements on cortical neuron activity suggest that our eye-tracking method might be used to account for some fraction of the variability in cortical neuron responses [4] . Neural variability is typically gauged by comparing the spike train responses to repeated presentations of the same stimulus ( Fig. 7a ). For awake animals, however, the presence of fixational eye movements, which are different from trial-to-trial ( Fig. 7b ), can introduce variability in the retinal stimulus itself. Using the estimated model for an example parafoveal neuron ( Fig. 7c ), we can gauge the effects of such eye movements on its firing rate ( Fig. 7d ). Note that the standard approach is to treat all the across-trial variability in the neuron’s response as ‘noise’, but in this case the model-predicted firing rates on different trials (in response to the same displayed stimulus but eye position-dependent retinal stimuli) were largely dissimilar (average correlation <0.3). 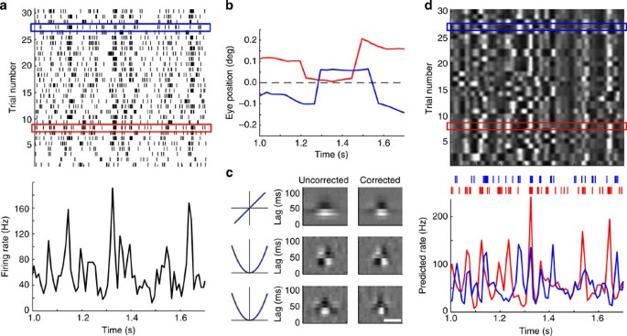Figure 7: The effects of eye movements on measures of cortical variability. (a) Spike raster for a parafoveal neuron (top; eccentricity 3.7°), in response to repeated presentations of a frozen noise stimulus, along with the across-trial average firing rate (PSTH; bottom). (b) Inferred eye positions are different on each trial: shown for two example trials (red and blue boxes ina). (c) The quadratic model for this neuron, estimated before (left) and after (right) correcting for the inferred eye positions. Horizontal scale bar is 0.25°. (d) As a result of the different eye positions on each trial, the model-predicted firing rates were highly variable across trials (top), predicting much of the trial-to-trial variability shown in the observed data (a). The model-predicted firing rates for the red and blue trials highlighted ina,dare shown below. Coloured tick marks above show the corresponding observed spike times. Figure 7: The effects of eye movements on measures of cortical variability. ( a ) Spike raster for a parafoveal neuron (top; eccentricity 3.7°), in response to repeated presentations of a frozen noise stimulus, along with the across-trial average firing rate (PSTH; bottom). ( b ) Inferred eye positions are different on each trial: shown for two example trials (red and blue boxes in a ). ( c ) The quadratic model for this neuron, estimated before (left) and after (right) correcting for the inferred eye positions. Horizontal scale bar is 0.25°. ( d ) As a result of the different eye positions on each trial, the model-predicted firing rates were highly variable across trials (top), predicting much of the trial-to-trial variability shown in the observed data ( a ). The model-predicted firing rates for the red and blue trials highlighted in a , d are shown below. Coloured tick marks above show the corresponding observed spike times. Full size image By decomposing these predicted firing rates into their across-trial average and eye movement-induced trial-to-trial fluctuations, we find that the latter account for nearly 70% of the overall variance. That these predicted trial-to-trial fluctuations are capturing real variability in the neuron’s response is demonstrated by the fact that they provide a 2.6-fold improvement in R 2 compared with the trial-average prediction. In fact, the eye-corrected model prediction ( R 2 =0.24) substantially outperforms even the ‘oracle model’ given by the empirical trial-averaged firing rate (that is, the peri-stimulus time histogram (PSTH); R 2 =0.14). Because standard characterizations of variability using repeated stimuli implicitly assume that the stimulus-driven firing rate is the same across trials, such eye position-dependent variability will be mistakenly attributed to noise, suggesting the reliability of V1 responses may typically be underestimated [4] . Studies of high-acuity visual processing have been limited by the lack of eye-tracking methods with sufficient accuracy to control for fixational eye movements. Here, we present a method for high-resolution eye position inference based on the idea that visual neurons’ activity can be utilized to track changes in the position of the stimulus on the retina [5] , [29] , [30] . We utilize multi-electrode array recordings combined with recently developed probabilistic modelling techniques [21] , [22] , [23] , [24] to provide estimates of eye position with accuracy on the order of 1 min of arc. Our method also provides continuous estimates of eye position uncertainty, typically below 1 arc-min. Previous studies have also utilized hardware measurements of eye position to correct for fixational eye movements, with mixed degrees of success [3] , [4] , [5] , [6] , [35] , [38] . Although the accuracy of hardware-based eye-tracking methods will vary depending on experimental factors and preprocessing methods [5] , [6] , [9] , they are unlikely to provide sufficient accuracy for studying foveal V1 processing [5] , [9] ( Supplementary Fig. 2 ). Our model-based eye position inference procedure can also naturally incorporate such hardware-based measurements to provide additional evidence, and can thus augment hardware-based tracking to provide much higher accuracy. In cases not requiring gaze-contingent experimental control, including studies of the rodent visual system [39] , it may even be able to supplant the use of hardware trackers altogether. Likewise, our method could be used to track the slow drift, as well as heartbeat- and respiration-related movements, present in anaesthetized and paralysed animals [2] . Although we demonstrate our method primarily using recordings from a 96-electrode Utah array while presenting ‘random-bar’ stimuli, it can be applied to a much broader range of experimental conditions. First, our procedure is robust to the precise size and composition of the neural ensemble used ( Fig. 5 ), allowing for it to be applied with a range of multi-electrode configurations used in typical V1 experiments, including linear and planar electrode arrays. Second, it can be used with a wide range of dynamic noise stimuli (for example, two-dimensional Gabor noise; Fig. 4 ), and can in principle be extended to natural movies, with the primary consideration simply being how efficiently a given stimulus can be used to estimate stimulus processing models. Finally, the eye-tracking procedure is largely insensitive to the particular choice of stimulus processing models. Here we used quadratic models that can robustly describe the range of single- and multi-unit responses in V1. However, more intricate models can easily be incorporated into this framework, and—to the extent that they provide better descriptions of V1 stimulus processing—they will improve the performance of the eye-tracking method. The primary purpose of the eye-tracking procedure presented here is to allow the estimation of detailed functional models of foveal V1 neurons. In doing so, this method opens the door for detailed studies of foveal visual cortical processing, which will allow for direct experimental tests of a number of important questions regarding potential specialization of the structural organization, functional properties and attentional modulation of foveal visual processing [17] , [18] , [19] , [20] . In fact, a recent report showed that visual acuity is not uniform within the fovea [20] , suggesting that such specialization of processing might even exist within the foveal representation itself. Because the precision of our eye-tracking method scales with the RF sizes of the neurons being recorded, it could indeed be applied to study V1 neurons with even finer RFs than those studied here. In addition, by providing precise measurement of fixational eye movements concurrently with recordings of V1 activity, our method could be used to resolve ongoing debates about the precise nature of such eye movements, and their role in visual coding and perception [40] , [41] , [42] . However, the impact of this method extends beyond the estimation of stimulus processing models in the fovea. First, we show that, even for parafoveal neurons at >4° eccentricity, our method could provide >2-fold improvements in model performance, suggesting that such accurate eye tracking will have a significant impact on a majority of studies in awake primate V1. Second, our method can be used to determine the contribution of fixational eye movements to measures of cortical variability [4] ( Fig. 7 ). Given that fixational eye movements create trial-to-trial variability in the underlying retinal stimulus itself, they will also have a significant impact on measures of ‘noise correlations’ [25] , [26] , [27] . In particular, without accounting for fixational eye movements, estimates of neurons' noise correlations can be confounded by the similarity of their stimulus tuning (‘stimulus correlations’). Our method could thus be critical for accurately characterizing the magnitude and structure of cortical variability in awake animals, issues that have important implications for cortical coding more generally [25] , [26] , [27] . Electrophysiology Multi-electrode recordings were made from primary visual cortex (V1) of two awake head-restrained male rhesus macaques ( Macaca mulatta ; 13- to 14-years old). We implanted a head-restraining post and scleral search coils under general anaesthesia and sterile conditions [5] . Animals were trained to fixate for fluid reward. In one animal, we also implanted a 96-electrode planar ‘Utah’ array (Blackrock Microsystems; 400 μm spacing). In the second animal, we implanted a recording chamber and used a custom microdrive to introduce linear electrode arrays (U-probe, Plexon; 24 contacts, 50 μm spacing) on each recording day. Eye position was monitored continuously using scleral search coils in each eye, sampled at 600 Hz. Stimuli were displayed on cathode ray tube (CRT) monitors (100 Hz refresh rate) subtending 24.3 × 19.3° of visual angle, viewed through a mirror haploscope. All protocols were approved by the Institutional Animal Care and Use Committee and complied with Public Health Service policy on the humane care and use of laboratory animals. Broadband extracellular signals were sampled continuously at 30 or 40 kHz and stored to disk. Spikes were detected using a voltage threshold applied to the high-pass filtered signals (low cutoff frequency 100 Hz). Thresholds were set to yield an average event rate of 50 Hz, and were subsequently lowered if needed to capture any putative single-unit spiking. Spike sorting was performed offline using custom software. Briefly, spike clusters were modelled using Gaussian mixture distributions that were based on several different spike features, including principal components, voltage samples and template scores. The features providing the best cluster separation were used to cluster single units. Cluster quality was quantified using both the ‘L-ratio’ and ‘isolation distance’ [43] . Only spike clusters that were well isolated using these measures—confirmed by visual inspection—were used for analysis. Multi-units were defined as spikes detected on a given electrode that did not belong to a well-isolated single-unit cluster. In linear array recordings, the electrodes are close enough that single units on one probe frequently make a significant contribution to the multi-unit activity on adjacent probes. We therefore excluded single-unit spikes from multi-units on adjacent probes. Visual stimuli For one-dimensional eye position inference, we used a ternary bar noise stimulus, consisting of random patterns of black, white and grey bars (matching the mean luminance of the screen). For the linear array recordings, the orientation of the bars was chosen to correspond to the preferred orientation of the majority of units recorded in a given session. However, for the planar array—with electrodes spanning many orientation columns—we used horizontal bars. Bars stretched the length of the monitor, and had a width of 0.057° for the Utah array recordings, and ranged from 0.038° to 0.1° for the linear array recordings (yielding consistent results). Bar patterns were displayed at 100 Hz, and were uncorrelated in space and time. The probability of a given bar being non-grey (that is, black or white) was set to a sparse value in most experiments (88% grey), but some experiments used a dense distribution (33% grey), yielding similar results. In most cases, the stimuli presented to both eyes were identical and allowed for estimation of a single position for the left and right eyes, assuming perfect vergence. In a subset of cases, we presented binocularly uncorrelated stimuli, allowing for estimates of separate left and right eye positions. For two-dimensional eye position inference (performed during Utah array recordings), we used two different types of stimuli. The first was a simple extension of the one-dimensional stimulus described above, where frames with horizontal and vertical bars were randomly interleaved ( Fig. 4a ). The second stimulus consisted of randomly placed Gabors with random sizes, orientations and spatial phases, chosen from distributions that were scaled to cover the range of tuning properties observed for recorded neurons ( Fig. 4c ). The number of Gabors per frame was ‘sparse’, and randomly selected from a Poisson distribution. The interleaved bar patterns were presented at 100 Hz, and for the sparse Gabor stimulus, we used a frame rate of 50 Hz. Behavioural task The animals were required to maintain fixation near a small point for each four second trial in order to earn a liquid reward. In some experiments, the fixation point made periodic jumps (every 700 ms) and the animals were required to make saccades to the new fixation point location. In these cases, the new fixation point was located 3° in either direction along the long-axis of the bar stimuli, such that an accurate saccade to the new fixation point would not alter the retinal stimulus. In practice, the animals typically did not saccade exactly to the new fixation point, and would often make one or more corrective microsaccades shortly following the initial saccade. However, the magnitude of these errors, and the corrective microsaccades, were comparable to that of microsaccades observed during the static fixation task. We also verified that our results were similar when we restricted analysis to only those experiments where the fixation point was static. Estimation of stimulus models Given an estimate of the retinal stimulus, we construct a ‘time-embedded’ stimulus vector S ( t ), which incorporates the stimulus at time t , as well as a range of previous time steps. We then fit a model describing each neuron's spike probability r i ( t ) as a function of S ( t ). Because nonlinear stimulus processing is common in V1 neurons [36] , [44] , we utilize a recently developed modelling framework [21] , [22] , [23] , [24] that describes stimulus processing as a second-order linear-nonlinear (LN) cascade. Specifically, the spike probability of a neuron is given by a sum over LN subunits, followed by a spiking nonlinearity function: where the k j are a set of stimulus filters, with corresponding static nonlinearities f j (. ), the w j are coefficients that determine whether each input is excitatory or suppressive (constrained to be ±1), and F [.] is the spiking nonlinearity function. Note that we also include a linear filter h to model the effects of additional covariates X ( t ) that are important for explaining the firing rate. Specifically, we use X ( t ) to model changes in average firing rate over a long experiment as well as modulation by saccades/microsaccades [45] . These additional covariates enhance the ability of the particular models to explain the data, but are not required for the general method. For example, when inferring eye position over scales larger than fixational movements, one could incorporate the effects of eye position ‘gain-field’ modulation [46] by including additional covariates in the model containing polynomials in the (coarse) eye position coordinates [47] . Although the set of functions f j (.) can be inferred from the data [21] , [23] , [24] , in this case, we limit the f j (.) to be linear and squared functions, which represents a (low-rank) quadratic approximation of the neuron's stimulus-response function [22] that provides a robust description of the stimulus processing of V1 simple and complex cells [24] . The model for each neuron is then characterized by a parameter vector Θ containing the set of stimulus filters k j , input signs w j , linear filter h and any parameters associated with the spiking nonlinearity function F [.]. Here we use a spiking nonlinearity of the form: Assuming that the observed spike counts of the i th neuron R i ( t ) are Poisson distributed with mean rate r i (t), the log-likelihood (LL i ) of Θ i given R i ( t ) is (up to an overall constant) [48] , [49] : We also incorporate spatiotemporal smoothness and sparseness regularization on the stimulus filters. Details regarding stimulus filter regularization, as well as methods for finding maximum likelihood parameter estimates have been described previously [24] . Assuming that the spiking of an ensemble of N units at time t is conditionally independent given the stimulus, the joint LL( t ) of observing the spike count vector (across all neurons) R ( t )=[ R 1 ( t ) R 2 ( t ) … R N ( t )] is given by a sum over the individual neurons’ LLs: Latent variable model of eye position To estimate the animal’s eye position as a function of time, we introduce a latent variable Z ( t ), which can take one of K possible values at each time, representing a discrete set of eye positions relative to the fixation point. The goal is then to infer Z ( t ), along with the parameters Θ of the stimulus processing models, given the observed spiking of all neurons R ( t ). Here, we consider a scalar-valued latent variable (representing a single dimension of eye position); however, the generalization to vector-valued (two-dimensional, or binocular) eye position variables is done by simply including a second latent variable of the same form. Because each value of Z ( t ) corresponds to a translation of the stimulus matrix S ( t ), we can use equation (4) to compute p [ R ( t )| Z ( t ); Θ ] for each value of Z ( t ) directly. We model the latent state sequence Z ( t ) as a first-order Markov process whose dynamics are determined entirely by a state-transition matrix A , such that A xy = p [ Z ( t )= y | Z ( t −1)= x ]. We then use an EM algorithm to alternate between estimating the model parameters Θ given p [ Z ( t )], and estimating p [ Z ( t )] given Θ . We use the standard forward-backward algorithm to estimate p [ Z ( t )] given Θ (ref. 50 ). When estimating model parameters, we utilize point estimates of Z ( t ) (the posterior mean), rather than maximizing the expected log likelihood under p [ Z ( t )]: E p ( Z ) [ p ( R ( t )|Θ; Z (t))]. This corresponds to ‘hard’ or ‘classification’ EM [51] , and provides a fast and robust alternative to standard EM [52] . We find similar results when using the maximum a posteriori estimate of Z ( t ), rather than the posterior mean. We also use the posterior s.d. as a measure of uncertainty. Two-stage eye position estimation Our model for the dynamics of Z ( t ) is based on segregating eye movements into periods of slow drift and occasional saccadic jumps. This segregation (that is, detection of saccades/microsaccades) can be easily accomplished using standard eye-tracking hardware, such as scleral search coils and video trackers [9] , [45] , [53] . Given this segregation, an efficient approach is to first infer the average eye position within each fixation, and subsequently to estimate the within-fixation changes in eye position (drift). We refer to the former as fixation-corrections Z fix ( i ), where i indexes the fixation number, and the latter as drift corrections Z drift ( t ). Mapping fixation indices to time we have that Z ( t )= Z fix ( t )+ Z drift ( t ). As Z fix ( t ) accounts for most of the variability in Z ( t ), this results in a coarse-to-fine inference procedure. It is also possible to estimate Z ( t ) in a single stage, producing largely similar results, although it is more computationally intensive. Thus, we apply the EM algorithm first to iterate between estimating model parameters Θ and Z fix ( i ) until convergence. We then use our estimate of Z fix ( i ) to construct a corrected stimulus matrix, which we use to iteratively estimate Θ and Z drift ( t ). Although we use the same general procedure described above, the LL calculations and the state transition matrices are different for each of these stages. For the estimation of Z fix ( i ), the LL is computed over a range of possible fixation positions given by summing equation (4) over time within each fixation. We assume a prior for the set of fixation positions given by a Gaussian centred at the fixation point, which is implemented through the state transition matrix: Here the state transition matrix only depends on the eye position y within the current fixation, but it will be extended in the next section to incorporate information from eye-tracking hardware. When estimating Z drift ( t ), we impose the assumption that it varies slowly in time by using a Gaussian ‘prior’ on the change in eye position between adjacent time points: which can also be viewed as a zero-mean Gaussian prior on the instantaneous drift velocity. Because predicted firing rates r ( t ) of the neurons at time t depend on the recent history of the stimulus, the likelihood function will depend not only on Z drift ( t ) at time t , but also on its recent history. However, to maintain tractability, we assume that: which is reasonable given that Z drift ( t ) varies slowly in time. The LL typically converges after only a few iterations for both Z fix ( i ) and Z drift ( t ) ( Supplementary Fig. 4 ). Although the results of EM algorithms can often depend on their initialization [50] , [54] , we find that our estimates of Θ and Z are remarkably insensitive to their initialization. For example, when we randomly initialized Z fix ( i ) (rather than initializing them to zero), we attained nearly identical results ( Supplementary Fig. 4 ). Similarly, even when the initial estimates of Z ( t ) were very far from their true values, and the resulting initial estimates of Θ were very poor, the EM algorithm was able to recover accurate estimates of both (see Fig. 6c–e ). Incorporating eye coil measurements Although evidence from eye-tracking hardware could be incorporated in many different ways, we find that eye coils provide a relatively reliable measure of shorter timescale changes in eye position, such as saccade amplitudes and moment-to-moment drift. In contrast, they are much less reliable for recording absolute eye position [5] . Thus, when estimating Z fix ( i ), we can incorporate the measured changes in average eye position between adjacent fixations, Δ e ( i )= e ( i )− e ( i -1), by adding an addition term to the transition matrix above (equation 6): where σ 2 noise is the assumed noise variance of the measurement. Similarly, when estimating Z drift ( t ), we can also incorporate evidence from the measured change in eye position between adjacent time points so that the state-transition matrix at time t is given by: where , and . Note that σ noise is a different parameter in this case, characterizing the noise level of measurements of instantaneous drift. For our results that make comparisons between inferred and coil-measured eye positions, we do not use the eye coil signals (other than to detect saccade times). Furthermore, we also did not use the eye coil signals for recordings with the Utah array, where the 96 electrodes seemed to provide sufficient neural evidence that doing so did not further improve model performance. Reconstructing eye position from Z ( t ) Because the latent variable Z ( t ) represents a translation of the time-embedded stimulus matrix S ( t ), it corresponds to an estimate of eye position over the range of time lags represented by S ( t ). Although we have, strictly speaking, assumed that the eye position is constant over this time scale, Z ( t ) will be determined predominantly by the retinal stimulus over a narrow range of time lags where V1 neurons are most responsive to the stimulus. Indeed, most V1 neurons were strongly modulated by the stimulus at latencies from about 30 to 70 ms. Thus, to derive estimates of eye position, we simply shifted our estimates of Z ( t ) backwards in time by 50 ms. This backwards shift was applied within each fixation, where the eye position was only slowly varying in time because of drift. Note that this 50 ms temporal delay was also utilized when incorporating eye position measurements with the coils into the state-transition matrix . Thus, inferred jumps in Z ( t ) were assumed to occur 50 ms after the measured saccade times and so on. General analysis details All data analyses were performed at a time resolution equal to the frame duration of the stimulus: 10 ms for all analysis except the 2D Gabor noise stimulus, which was 20 ms. Only trials lasting at least 750 ms were used, and the first 200 ms and last 50 ms of each trial were excluded from analysis to avoid effects due to onset transients, fixation breaks or blinks. Multi-units and single-units were selected for analysis based on the cross-validated LL of their initial model fits (before estimating eye position). Only those units that had cross-validated LL values greater than 0 were used in the analysis. This choice (which excluded<5% of units) was implemented primarily to eliminate noisy multi-unit channels, although such ‘uninformative’ units are naturally ignored by the algorithm because they provide very little evidence for particular eye positions. We used a lattice representing a range of possible values for Z fix spanning about ±0.85°, and for Z drift spanning about ±0.45°. In most cases, we used a lattice spacing of about Δ Z =0.03°, although we also ran a final iteration of estimating eye position using a higher resolution of Δ Z =0.015° to allow for more precise comparisons with the eye coil data. Although most analyses were performed at the base time resolution specified above, for inferring drift we used a slightly lower time resolution Δ t drift and linearly interpolated the eye positions between these time points. This is equivalent to assuming that the drift velocity is piecewise constant over a time scale Δ t drift , and ensures that neural activity can provide sufficient evidence for a change in eye position Δ Z . We found that Δ t drift of two or three times the base temporal resolution (20 or 30 ms) provided good results. As described above, the state-transition matrices for Z fix and Z drift were governed by the parameters σ fix and σ drift , respectively. The choice of σ fix controls the bias towards small deviations from the fixation point, whereas σ drift controls the smoothness of the inferred drift. Likewise, the σ noise parameters determine the relative weight given to evidence provided by eye-tracker measurements. We set these parameters heuristically to produce smooth inferred eye positions that captured much of the dynamics measured with the eye coils, although we find similar results over a range of values for these parameters. The entire iterative estimation procedure could be performed in a matter of hours on a desktop personal computer (Intel core i7 processor, 3.30 GHz × 6; 64 GB RAM). Specifically, with a recording from the Utah array consisting of about 100 units, our procedure took around 5 min to run per minute (6,000 samples) of data. Note that a majority of this time was usually spent estimating the parameters of the stimulus models, which depends on the nature of the stimulus and the structure of the models [24] . A Matlab implementation of our algorithm can be downloaded from http://www.clfs.umd.edu/biology/ntlab/EyeTracking . Statistical analyses Unless otherwise stated, we used robust statistics as our data were often strongly non-Gaussian (with heavy tails). Paired comparisons of group medians were performed with two-sided Wilcoxon signed rank tests. Correlations were computed using the nonparametric Spearman’s rank correlation. Linear regression analysis was performed using Matlab’s robust regression routine. We use a robust estimate of the standard deviation based on the median absolute deviation, given by: Note that the scaling factor of 1.48 is used to provide an estimate of variability that converges to the standard deviation for a normal distribution. The use of a robust estimate of variability was particularly important when analysing distributions of the differences between two eye position estimates, which were often sharply peaked at zero, while exhibiting occasional large deviations. Other robust estimates of variability, such as the inter-quartile range, gave qualitatively similar results. Quantifying stimulus filter properties The spatial tuning properties of each unit were quantified using several measures, including the spatial envelope width, spatial frequency and filter amplitude. Specifically, for each stimulus filter, we fit a Gabor function to its spatial profile at the best latency (defined as the latency with highest spatial variance): The envelope width was defined as 2 σ , the spatial frequency was given by 1/ λ and the filter amplitude was given by α . These numbers were computed for each filter before and after correcting for eye position. We separately report values for the linear filter, and the best squared filter for each unit (although one SU did not have a resolvable squared filter). When computing the overall RF width of each neuron ( Fig. 6 ), we used a weighted average of the RF widths of the individual filters, weighted by the strength of each filter’s contribution to the overall response of the neuron. When computing model properties across all units ( Fig. 6a,b ), we excluded a small fraction of units (7/357) because of poor model fits (4/357) or because a discontinuous change in RF positions with electrode depth suggested the deepest probes were positioned in a separate patch of cortex (3/357). Results were nearly identical without exclusions of these units. To quantify the degree to which neurons exhibited linear ‘simple-cell-like’ stimulus processing versus spatial-phase invariant ‘complex-cell-like’ processing, using responses to ternary bar stimuli, we defined a measure of spatial phase sensitivity termed the phase-reversal modulation. It is defined as the average difference between the responses to a stimulus and its inverse, normalized by the overall average rate, and is given by: where r [ S ( t )] is the predicted response to the stimulus at time t , r [− S ( t )] is the predicted response to the polarity-reversed stimulus and is the average rate. It thus measures the sensitivity of a neuron to the spatial phase of the stimulus, similar to the standard ‘F1/F0’ measure used with drifting grating stimuli [33] . Measuring model performance To quantify the goodness-of-fit of our models, we use the likelihood-based ‘pseudo- R 2 ’ (refs 34 , 55 ), defined as: where LL model , LL full and LL null are the LLs of the estimated model, the ‘full’ model and the ‘null’ model, respectively. In our case, the null model included any covariates other than the stimulus. This likelihood-based R 2 measure is analogous to the standard coefficient of determination for more general regression models, and is identical to it when using a Gaussian likelihood function. It can also be related to measures of information conveyed by a neuron’s spiking about the stimulus [21] , [56] . Note that pseudo- R 2 describes the ability of a model to predict neural responses on single trials, rather than trial-average responses where a Gaussian noise model can be used, which is a key feature of analysing the responses in the presence of fixational eye movements where the retinal stimulus cannot be controlled/repeated. To quantify changes in model performance, we report the ratio of R 2 after correcting for eye position to its value before correcting for eye position. To avoid problems with over-fitting, we used a ‘leave-one-out’ cross-validation procedure to estimate the model parameters (and evaluate model performance) of each unit. Thus, for each of N units in a given recording, the entire iterative procedure for estimating eye position and the stimulus models was repeated, excluding the activity of that unit. The resulting eye position estimates were used to fit model parameters and measure model performance for the excluded unit. Analysing eye coil signals Measurements of eye position relative to the fixation point were median-subtracted within each recording block, and were calibrated to remove any linear relationships between horizontal and vertical positions. Saccades were detected as times when the instantaneous eye velocity exceeding 10° s −1 , and microsaccades were defined as saccades whose amplitude was less than 1° (refs 45 , 53 ). When comparing inferred and measured microsaccade amplitudes, we excluded any detected microsaccades where the preceding or subsequent fixation lasted less than 100 ms. When comparing inferred and measured drift, we only used fixations lasting longer than 150 ms. For the first monkey (used for the Utah array recordings), one of the eye coils was found to be unreliable and was thus excluded from all analysis. For the second monkey (used for the linear array recordings), we used the average position over both eye coils, which yielded a more reliable signal. Simulating neural ensembles with different RF sizes To determine how our eye position inference procedure depends on the RF sizes of the neurons used, we simulated populations of neurons similar to those observed with the array, but having different RF sizes. Specifically, we used the set of stimulus models obtained (after inferring eye positions) from an example Utah array recording, and applied a uniform spatial scaling factor (ranging from 0.25 to 4) to the stimulus filters of all units, as well as to the bar stimuli used. The resulting average RF widths thus range from 0.03° to 0.48°. We then simulated firing rates for each neural model in response to the stimulus during a particular ‘ground-truth’ sequence of eye positions (generated from the eye position estimates of our model from an example recording). We used these simulated firing rates to generate Poisson distributed spike counts. Given these ‘observed’ spike counts, we applied our algorithm to estimate the eye position sequence, and the stimulus filters of the model neurons. We verified that the ability of the model to find the ‘ground truth’ eye positions ( Supplementary Fig. 1 ) did not depend on using a particular simulated eye position sequence, and we obtained similar results for other eye position sequences, such as those based on the eye coil measurement. Effects of eye movements on cortical variability For analysis of cortical variability ( Fig. 7 ), we performed an experiment where the same ‘frozen noise’ stimulus was presented on a subset of trials, randomly interleaved with other non-repeating stimulus sequences. These ‘repeat’ trials were not used for training the stimulus models. The inter-trial variability of cortical responses due to eye movements was quantified by evaluating the firing rate predicted by the stimulus model on each trial, given the inferred eye position sequences. Treating the sequence of firing rates predicted on each trial as a vector, we computed several measures of eye movement-induced trial-to-trial variability, including the average correlation between single-trial firing rates: where ρ ( r i , r j ) is the Spearman’s rank correlation between the firing rate vector in the i th and j th trials, and the average is computed across pairs of unique trials. We also compute the fraction of total variability accounted for by across-trial variation as: How to cite this article: McFarland, J. M. et al . High-resolution eye tracking using V1 neuron activity. Nat. Commun. 5:4605 doi: 10.1038/ncomms5605 (2014).